In situ tuning of electronic structure of catalysts using controllable hydrogen spillover for enhanced selectivity In situ tuning of the electronic structure of active sites is a long-standing challenge. Herein, we propose a strategy by controlling the hydrogen spillover distance to in situ tune the electronic structure. The strategy is demonstrated to be feasible with the assistance of CoO x /Al 2 O 3 /Pt catalysts prepared by atomic layer deposition in which CoO x and Pt nanoparticles are separated by hollow Al 2 O 3 nanotubes. The strength of hydrogen spillover from Pt to CoO x can be precisely tailored by varying the Al 2 O 3 thickness. Using CoO x /Al 2 O 3 catalyzed styrene epoxidation as an example, the CoO x /Al 2 O 3 /Pt with 7 nm Al 2 O 3 layer exhibits greatly enhanced selectivity (from 74.3% to 94.8%) when H 2 is added. The enhanced selectivity is attributed to the introduction of controllable hydrogen spillover, resulting in the reduction of CoO x during the reaction. Our method is also effective for the epoxidation of styrene derivatives. We anticipate this method is a general strategy for other reactions. Highly efficient and selective catalysts are important for the industrial production of commodity chemicals, as well as fine chemicals and pharmaceuticals [1] . The development of new heterogeneous catalysts for carrying out multipath reactions with high selectivity to achieve high-yield production of target chemicals is a longstanding challenge [2] , [3] . The final product distribution, i.e., the selectivity of a reaction over a given catalyst, is determined by the relative activation barrier among different reaction paths, which in nature, primarily depend on the electronic structure of the catalytic active sites [4] , [5] , [6] . However, under reaction conditions, the electronic structures of active sites are easily affected by temperature, atmosphere, and absorbed species [7] , [8] . It is difficult to control the active sites to maintain the optimal electronic structure during the reaction, which favors producing more target products. Some researchers have devoted substantial effort to studying how to control and tune the electronic structures of the active sites responsible for activity and selectivity under real reaction conditions [9] , [10] . In contrast to numerous studies on identifying catalytically active sites under real-time reaction conditions [11] , [12] , [13] , [14] , limited methods have been reported for controlling and tuning the electronic structure of active sites during a reaction. In general, the hydrogen migration from the metal particles to the support, i.e., hydrogen spillover, is a well-known phenomenon in heterogeneous catalysis and is involved in many important reactions [15] , [16] , [17] , [18] , [19] , [20] , [21] , [22] , [23] , [24] . The efficiency and spatial extent of hydrogen spillover strongly depend on the types of supports [25] , [26] . For instance, a well-defined model system demonstrated that on the nonreducible alumina support, hydrogen spillover is limited to short distances, with the hydrogen flux decreasing over distance to create a concentration gradient [25] . In-depth understanding of hydrogen spillover can not only help to explain experimental phenomena but also aid the design of advanced catalysts with enhanced catalytic performances [27] , [28] , [29] , [30] , [31] , [32] , [33] , [34] , [35] . Being inspired by these researches, we posit that there is an opportunity for an approach to modulating the electronic structure of active sites through regulating hydrogen spillover strength for enhanced catalytic performance. In this work, using the CoO x catalyzed epoxidation reaction of styrene as an example, we propose an approach to tune the electronic structure of cobalt species during the reaction by the introduction of controllable hydrogen spillover, to enhance the selectivity of styrene oxide (SO). To demonstrate the strategy, a CoO x /Al 2 O 3 /Pt catalyst is prepared by a facile and general template-assisted atomic layer deposition (ALD) method [36] , [37] , [38] , in which CoO x and Pt nanoparticles are attached on the outer and inner surfaces of Al 2 O 3 nanotubes, respectively. The strength of hydrogen spillover from Pt to CoO x can be precisely tailored by varying the thickness of the Al 2 O 3 layer. The CoO x /Al 2 O 3 /Pt catalyst with 7 nm-thick Al 2 O 3 layer exhibits greatly enhanced selectivity (from 74.3% to 94.8%) when H 2 atmosphere is introduced. Detailed analyses reveal that the cobalt species under the oxidation condition are reduced to a lower oxidation state by introducing the controllable hydrogen spillover, leading to a higher SO selectivity. Synthesis and characterization of the catalysts CoO x / y Al 2 O 3 /Pt catalysts with a separating Al 2 O 3 layer were obtained using carbon nanocoils (CNCs) as sacrificial templates (Supplementary Fig. 1 ). First, Pt nanoparticles and an Al 2 O 3 layer were deposited onto CNCs by Pt ALD and Al 2 O 3 ALD, respectively. Subsequently, the CNC templates were removed by calcination under ambient atmosphere. Finally, CoO x nanoparticles were deposited by CoO x ALD, producing CoO x / y Al 2 O 3 /Pt (where y is the cycle numbers of ALD Al 2 O 3 ). For comparison, two reference catalysts (CoO x /50Al 2 O 3 and 50Al 2 O 3 /Pt) were also synthesized by a similar method. 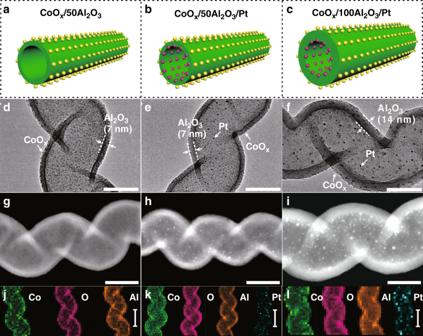Fig. 1: Structural characterization of the catalysts. a–cStructure diagrams (The green tubes represent Al2O3. The magenta and yellow balls represent Pt and CoOx, respectively),d–fTEM images (scale bar, 50 nm),g–iHAADF-STEM images (scale bar, 50 nm), andj–lEDX elemental mappings (scale bar, 100 nm) of the catalysts.a,d,g,j: CoOx/50Al2O3;b,e,h,k: CoOx/50Al2O3/Pt; andc,f,i,lCoOx/100Al2O3/Pt. Figure 1a–c present the structure diagrams of CoO x /50Al 2 O 3 , CoO x /50Al 2 O 3 /Pt, and CoO x /100Al 2 O 3 /Pt. Figure 1d–f show transmission electron microscopy (TEM) images of the three catalysts. TEM images of other catalysts, including CoO x / y Al 2 O 3 /Pt with different cycles of ALD Al 2 O 3 (35, 65, 80, and 300) and the reference catalyst (50Al 2 O 3 /Pt), are shown in Supplementary Fig. 2 . For all TEM images, Al 2 O 3 hollow structures can be clearly observed. The CoO x / y Al 2 O 3 /Pt with different Al 2 O 3 cycles (35, 50, 65, 80,100, and 300) possess varied Al 2 O 3 thicknesses from 5, 7, 9, 11, 14, to 41 nm. Regardless of Al 2 O 3 thicknesses, the outer CoO x and the inner Pt nanoparticles have similar average diameters (Supplementary Figs. 3 and 4 ), which is consistent with X-ray diffraction (XRD) result (Supplementary Fig. 7 and Supplementary Table 1 ). A high-resolution TEM (HRTEM) image of CoO x /50Al 2 O 3 /Pt is shown in Supplementary Fig. 5 . The high-angle annular dark field scanning transmission electron microscopy (HAADF-STEM) images (Fig. 1h, i ) of CoO x /50Al 2 O 3 /Pt and CoO x /100Al 2 O 3 /Pt clearly show that Pt nanoparticles are confined in Al 2 O 3 nanotubes. Energy-dispersive X-ray spectroscopy (EDS) mappings of the catalysts show that the distributions of Co, O, Al, and Pt (Fig. 1j and l) are consistent with the positions of the CoO x , Al 2 O 3 , and Pt layers. Further, the distributions of Co, Al, and Pt in CoO x /50Al 2 O 3 /Pt were revealed clearly by STEM image and EDX mapping (Fig. 2a–d ) of a cross-sectional specimen, prepared by focused ion beam (FIB) milling along the vertical direction of the Al 2 O 3 nanotubes. The line-scanning profile (Fig. 2e ) of cross-sectional composition shows that the signal of Co species was not detected in the Al 2 O 3 nanotubes, which clearly demonstrates the separated structure of CoO x /50Al 2 O 3 /Pt. The Al peak at ~4.5 nm is ascribed to signal of powder (from the FIB ion milling) remained in the space nearby the outer surface of the sample (Supplementary Fig. 6 ). 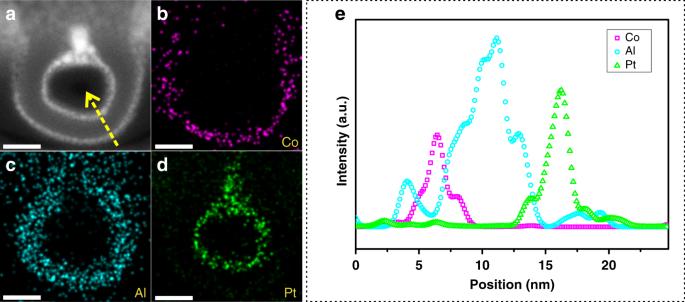Fig. 2: Structural characterization of CoOx/50Al2O3/Pt. aSTEM image (scale bar, 20 nm) andb–dEDX elemental mappings (scale bar, 20 nm) of a cross-sectional specimen of CoOx/50Al2O3/Pt prepared by focused ion beam milling.eCompositional point profile of Co, Al, and Pt from the specimen recorded along the yellow arrow shown ina. The Co and Pt contents in the catalysts, measured by inductively coupled plasma-atomic emission spectrometry (ICP-AES), are shown in Supplementary Table 2 . N 2 sorption experiments (Supplementary Fig. 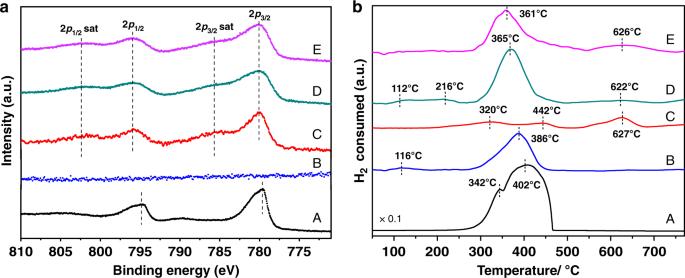Fig. 3: Electronic structure and chemisorption characterizations. aXPS Co 2panalysis andbH2-TPR profiles of (A) Co3O4as reference, (B) 50Al2O3/Pt, (C) CoOx/50Al2O3, (D) CoOx/50Al2O3/Pt, and (E) CoOx/100Al2O3/Pt. 8 and Supplementary Table 3 ) demonstrate that all the catalysts possess similar average pore diameter, while their Brunauer–Emmett–Teller (BET) surface areas and pore volumes increase with the decrease of Al 2 O 3 thicknesses. Fig. 1: Structural characterization of the catalysts. a – c Structure diagrams (The green tubes represent Al 2 O 3 . The magenta and yellow balls represent Pt and CoO x , respectively), d – f TEM images (scale bar, 50 nm), g – i HAADF-STEM images (scale bar, 50 nm), and j – l EDX elemental mappings (scale bar, 100 nm) of the catalysts. a , d , g , j : CoO x /50Al 2 O 3 ; b , e , h , k : CoO x /50Al 2 O 3 /Pt; and c , f , i , l CoO x /100Al 2 O 3 /Pt. Full size image Fig. 2: Structural characterization of CoO x /50Al 2 O 3 /Pt. a STEM image (scale bar, 20 nm) and b – d EDX elemental mappings (scale bar, 20 nm) of a cross-sectional specimen of CoO x /50Al 2 O 3 /Pt prepared by focused ion beam milling. e Compositional point profile of Co, Al, and Pt from the specimen recorded along the yellow arrow shown in a . Full size image X-ray photoelectron spectroscopy (XPS) results (Fig. 3a ) reveal the coexistence of Co 3+ and Co 2+ . Compared to the spinel Co 3 O 4 , the main 2 p peaks of CoO x /50Al 2 O 3 , CoO x /50Al 2 O 3 /Pt, and CoO x /100Al 2 O 3 /Pt shift to higher binding energy (the 2 p 3/2 peaks shift from 779.5 to 780.0 eV and the 2 p 1/2 peaks shift from 794.7 to 795.9 eV), and the satellite peaks appear (785.6 eV (2 p 3/2 sat) and 802.3 eV (2 p 3/2 sat)), indicating that the as-prepared CoO x nanoparticles consist of both Co 2+ and Co 3+ species [39] , [40] . Hydrogen temperature-programmed reduction (H 2 -TPR) was also employed (Fig. 3b ). Compared to CoO x /50Al 2 O 3 , the peak intensity of CoO x /50Al 2 O 3 /Pt centered at 622 °C decreases significantly, which is because the CoO x species can be additionally reduced by the spilled active hydrogen from Pt nanoparticles. The peak intensity of CoO x /100Al 2 O 3 /Pt centered at 626 °C is remained, possibly because the Al 2 O 3 layer of 100 ALD cycles (14 nm) is too thick and the hydrogen spillover effect is greatly weakened. 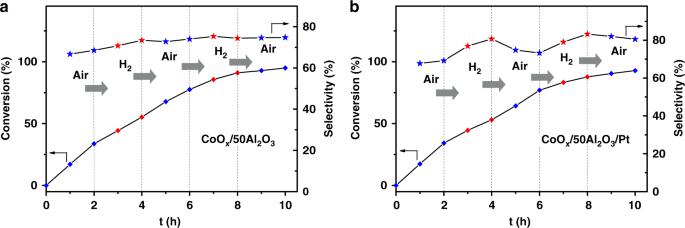Fig. 4: H2pulse experiments. The evolution of styrene conversion and SO selectivity with reaction atmosphere and time overaCoOx/50Al2O3andbCoOx/50Al2O3/Pt. The differences in reducibility of Co (Supplementary Table 4 ) demonstrate that the flux of spilled hydrogen species on the nonreducible Al 2 O 3 support decreases with increasing distance. Fig. 3: Electronic structure and chemisorption characterizations. a XPS Co 2 p analysis and b H 2 -TPR profiles of (A) Co 3 O 4 as reference, (B) 50Al 2 O 3 /Pt, (C) CoO x /50Al 2 O 3 , (D) CoO x /50Al 2 O 3 /Pt, and (E) CoO x /100Al 2 O 3 /Pt. Full size image Catalytic performance The epoxidation of olefins is an important chemical reaction since epoxides are key intermediates in organic synthesis [41] , [42] . The catalytic performances of different catalysts for the styrene epoxidation reaction with tert-butyl hydroperoxide (TBHP) as the oxidant are summarized in Table 1 . Styrene was negligibly converted without a catalyst (Table 1 , entry 1). For 50Al 2 O 3 /Pt, only a 17.7% conversion was obtained (Table 1 , entry 2). When Co-based catalysts were added, SO was formed as the major product, and benzaldehyde (BzH) was produced as a byproduct. For CoO x /50Al 2 O 3 , the reaction can be efficiently catalyzed, with 93% conversion and 74.3% SO selectivity (Table 1 , entry 3). All of the attempts, including the pre-reduction treatment (Table 1 , entry 4), the increase of the ratio of TBHP/styrene (Supplementary Fig. 9 ), the addition of a Pt component to the catalyst (namely CoO x /50Al 2 O 3 /Pt) (Table 1 , entry 6), and the introduction of H 2 into the reaction system (H 2 -TBHP) (Table 1 , entry 5), failed to enhance the SO selectivity of CoO x /50Al 2 O 3 . However, when H 2 was introduced into the reaction, the SO selectivity (94.8%) of CoO x /50Al 2 O 3 /Pt in the H 2 -TBHP condition (Table 1 , entry 7) was remarkably increased by 20.5% compared to CoO x /50Al 2 O 3 in the TBHP condition. Although its conversion (82.5%) was slightly reduced, the decreased conversion was easily compensated by prolonging the reaction time. During the entire reaction process, the SO selectivity of the CoO x /50Al 2 O 3 /Pt in the H 2 -TBHP condition is greatly higher compared with that of the CoO x /50Al 2 O 3 in the TBHP condition under the same styrene conversion (Supplementary Fig. 10 ). After reaction, the distributions of the inner Pt and the outer CoO x nanoparticles for CoO x /50Al 2 O 3 /Pt remain (Supplementary Fig. 11 ), and no obvious detachment of nanoparticles is observed, indicating that the catalyst is stable during the reaction. Table 1 Catalytic performances of the catalysts for styrene epoxidation reaction in different conditions a . Full size table Further, H 2 pulse experiments were carried out for CoO x /50Al 2 O 3 and CoO x /50Al 2 O 3 /Pt with alternating pulse of H 2 and air (Fig. 4a, b ). During the reaction, for CoO x /50Al 2 O 3 , the conversion and selectivity were almost unaffected by the alternate reaction atmosphere. For CoO x /50Al 2 O 3 /Pt, when air was displaced by H 2 , the increase of conversion slowed down and the SO selectivity was increased obviously. When H 2 was displaced by air, the opposite phenomenon occurred. This control experiment straightforwardly indicates that the introduction of active hydrogen (Pt and H 2 ) plays an essential role in enhancing the selectivity of the catalysts for styrene epoxidation reaction. Fig. 4: H 2 pulse experiments. The evolution of styrene conversion and SO selectivity with reaction atmosphere and time over a CoO x /50Al 2 O 3 and b CoO x /50Al 2 O 3 /Pt. 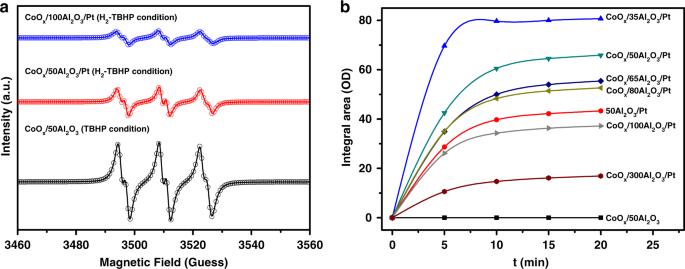Fig. 5: Catalytic mechanism analyses. aExperimental EPR spectra (lines) and simulated spectra (open circles) for a mixture of PBN–OOC(CH3)3and PBN–OC(CH3)3.bIntensity of the ʋ(OD) band during exposure of samples in (D2:H2= 1:1) at a total D2/H2flow rate of 30 ml min−1at 80 °C and 1 atm. Full size image The effect of the distance between CoO x and Pt components corresponding to the thicknesses of the Al 2 O 3 layer on the catalytic performance has been investigated (Table 2 and Supplementary Table 5 ). The thicknesses of the Al 2 O 3 layer are precisely regulated by varying the cycle numbers of ALD Al 2 O 3 . In TBHP condition, the catalytic performances of CoO x / y Al 2 O 3 /Pt are similar. However, when H 2 was introduced, their catalytic performances exhibited obvious differences. Varying the cycle numbers of ALD Al 2 O 3 from 35 to 65, the activities of the three catalysts in the H 2 -TBHP condition decreased compared with those of the corresponding catalysts in the TBHP condition, whereas the SO selectivities show obvious improvements with the highest value of 94.8% for CoO x /50Al 2 O 3 /Pt (Table 2 , entries 1–3). With a further increase of cycle numbers (over 80), the activities and SO selectivities of CoO x /80Al 2 O 3 /Pt, CoO x /100Al 2 O 3 /Pt, and CoO x /300Al 2 O 3 /Pt in the H 2 -TBHP condition are similar to that of the corresponding catalysts in the TBHP condition (Table 2 , entries 4–6). At low conversions, CoO x /50Al 2 O 3 /Pt catalyst also exhibits the greatest improvement of SO selectivity among these catalysts (Supplementary Fig. 12 ). Therefore, it can be seen that a precisely controlled CoO x –Pt distance is critically important for the remarkably enhanced SO selectivity. Table 2 Catalytic performances of the catalysts with different Al 2 O 3 cycles for styrene epoxidation reaction. Full size table Catalytic mechanism To uncover the potential mechanism for the enhanced SO selectivity, a series of experiments and characterizations were carried out. Isotope-labeling experiments were conducted to track the transfer pathways of split hydrogen species. For CoO x /50Al 2 O 3 /Pt in the D 2 -TBHP condition, the deuterium signal was not found in the mass spectrometry results of BzH and SO (Supplementary Fig. 13 ), demonstrating that the active hydrogen species were not directly involved in the oxidation of organic substrates. A free radical scavenger (butylated hydroxytoluene, BHT) was added to the reaction to further study the reaction mechanism. For CoO x /50Al 2 O 3 in the TBHP condition, and CoO x /50Al 2 O 3 /Pt and CoO x /100Al 2 O 3 /Pt in the H 2 -TBHP condition, the conversion of styrene stopped after the addition of BHT (Supplementary Fig. 14 ), indicating that the radical pathway has an important contribution to the reaction mechanism. Moreover, according to the electron paramagnetic resonance (EPR) results (Fig. 5a , Supplementary Fig. 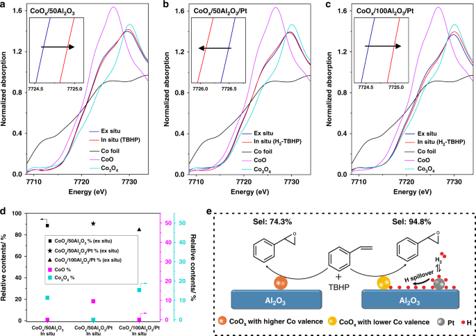Fig. 6: XANES spectra of the catalysts and proposed mechanisms. a–cEx situ and in situ Co K-edge XANES spectra of CoOx/50Al2O3, CoOx/50Al2O3/Pt, and CoOx/100Al2O3/Pt, and spectra of reference samples (Co foil, CoO, and Co3O4). Insets show the expanded sections of absorption edges.dThe results of the linear combination fitting for the in situ spectra of the catalysts. For each catalyst, the in-situ spectrum is fitted by a linear combination of the ex-situ spectrum and the spectra of reference samples (Co3O4and CoO).eProposed reaction mechanisms for CoOx/50Al2O3in the TBHP condition and CoOx/50Al2O3/Pt in the H2-TBHP condition. In the presence of controllable hydrogen spillover, cobalt species with a lower valence state are beneficial to the enhanced selectivity. 15 , and Supplementary Table 6 ), two kinds of radicals, i.e., tert-butylperoxy and tert-butyloxy radicals (tBuOO∙ and tBuO∙), can be detected in the three cases. These results indicate that the styrene epoxidation reaction over Co-based catalysts experienced a radical process, and the kinds of the radicals were the same in the three cases. Fig. 5: Catalytic mechanism analyses. a Experimental EPR spectra (lines) and simulated spectra (open circles) for a mixture of PBN–OOC(CH 3 ) 3 and PBN–OC(CH 3 ) 3 . b Intensity of the ʋ(OD) band during exposure of samples in (D 2 :H 2 = 1:1) at a total D 2 /H 2 flow rate of 30 ml min −1 at 80 °C and 1 atm. Full size image The existence of hydrogen spillover from Pt to CoO x through the nonreducible Al 2 O 3 support was confirmed by H–D exchange experiments (Fig. 5b and Supplementary Fig. 16 ). Figure 5b shows the H–D exchange rates of CoO x /50Al 2 O 3 , 50Al 2 O 3 /Pt, and CoO x / y Al 2 O 3 /Pt ( y = 35, 50, 65, 80, 100, and 300), indicating that the flux of spilled deuterium species from Pt to CoO x on the nonreducible Al 2 O 3 support decreases with increasing distance. The hydrogen spillover was also confirmed by the color change in the mixture of the catalyst and WO 3 nanowires (Supplementary Fig. 17 ). There are debates on the existence of hydrogen spillover on nonreducible support (SiO 2 , Al 2 O 3 , and zeolite). It was argued that hydrogen spillover to defect-free surfaces of nonreducible metal oxides cannot take place, but spillover to a non-reducible support with defects is possible [16] . In recent years, more and more evidence demonstrates that although Al 2 O 3 is a non-reducible oxide, hydrogen spillover can occur on it [25] , [43] , [44] , [45] , [46] , [47] , [48] , [49] . In this work, the obtained Al 2 O 3 is amorphous (Supplementary Fig. 7 ) and thus many defects exist. The nonreducible Al 2 O 3 support was calcined at high temperature, which may result in the formation of a small amount of micropores [50] . Thus, the active hydrogen species may spill over the surface of the micropores or through the defects of Al 2 O 3 layer. To reveal the electronic structures of cobalt species, X-ray absorption fine structure (XAFS) of the catalysts was investigated (Fig. 6a–c ). The ex situ X-ray absorption near-edge structure (XANES) profiles show that the positions of the white line peaks for the CoO x /50Al 2 O 3 , CoO x /50Al 2 O 3 /Pt, and CoO x /100Al 2 O 3 /Pt are all located between the peaks of the rock-salt CoO and spinel Co 3 O 4 , indicating that the oxidation states of cobalt species for as-prepared catalysts include both Co 3+ and Co 2+ , which is consistent with the XPS result. In the presence of TBHP, compared with the ex situ spectrum, the absorption edge of the in-situ spectrum for CoO x /50Al 2 O 3 shifted to higher energy (Fig. 6a ), revealing that the cobalt species in the reaction is at a higher oxidation state. The changes in the valence of catalyst are not significant, because of the mild reaction conditions (80 °C and atmosphere pressure). When H 2 was introduced into the reaction system, no obvious difference was observed in the H 2 -TBHP condition compared with in the TBHP condition for CoO x /50Al 2 O 3 (Supplementary Fig. 18 ). For CoO x /100Al 2 O 3 /Pt, a distinct increase in the cobalt oxidation state was also observed in the reaction (H 2 -TBHP condition) (Fig. 6c ). However, for CoO x /50Al 2 O 3 /Pt, the absorption edge of the in-situ spectrum shifted to lower energy (Fig. 6b ), meaning a decrease in the cobalt oxidation state in the H 2 -TBHP condition. To quantitatively reveal the change in the cobalt oxidation states during the reaction, the in-situ XANES spectrum is simulated by a linear combination of the ex-situ spectrum of the as-prepared catalyst and the spectra of reference samples (Co 3 O 4 and CoO) (Supplementary Fig. 19 and Supplementary Table 7 ). For CoO x /50Al 2 O 3 in the TBHP condition and CoO x /100Al 2 O 3 /Pt in the H 2 -TBHP condition, extra Co 3 O 4 (11.4% and 15.4%, respectively) is formed, as shown in Fig. 6d . However, for CoO x /50Al 2 O 3 /Pt in the H 2 -TBHP condition, extra CoO (9.6%) is formed. The k 2 -weighted Fourier-transformed extended X-ray absorption fine structure (FT-EXAFS) spectra (Supplementary Fig. 20 ) and their curve fitting results (Supplementary Table 8 ) are consistent with the conclusions drawn from the XANES experiments. Fig. 6: XANES spectra of the catalysts and proposed mechanisms. a – c Ex situ and in situ Co K-edge XANES spectra of CoO x /50Al 2 O 3 , CoO x /50Al 2 O 3 /Pt, and CoO x /100Al 2 O 3 /Pt, and spectra of reference samples (Co foil, CoO, and Co 3 O 4 ). Insets show the expanded sections of absorption edges. d The results of the linear combination fitting for the in situ spectra of the catalysts. For each catalyst, the in-situ spectrum is fitted by a linear combination of the ex-situ spectrum and the spectra of reference samples (Co 3 O 4 and CoO). e Proposed reaction mechanisms for CoO x /50Al 2 O 3 in the TBHP condition and CoO x /50Al 2 O 3 /Pt in the H 2 -TBHP condition. In the presence of controllable hydrogen spillover, cobalt species with a lower valence state are beneficial to the enhanced selectivity. Full size image Our results show that epoxidation selectivity can be obviously enhanced after controllable hydrogen spillover was introduced. The possible reasons of the enhanced selectivity were revealed by detailed experiments and characterizations. After Pt and H 2 were introduced into the epoxidation reaction, the CoO x catalyzed epoxidation reaction still experienced a radical process and the kinds of radicals were the same, which can be concluded from the radical scavenging and EPR results. On the other hand, for CoO x / y Al 2 O 3 /Pt, they are similar in sizes of nanoparticles (TEM and XRD) and pore diameter (N 2 sorption) regardless of the thicknesses of Al 2 O 3 . Their catalytic performances are similar in TBHP condition. Moreover, the pre-reduction treatment of CoO x /50Al 2 O 3 further indicates the enhanced selectivity is not ascribed to the ex-situ oxidation states of fresh catalysts. In contrast, when H 2 was introduced into the reaction, the catalytic performances of the CoO x / y Al 2 O 3 /Pt with different Al 2 O 3 thicknesses exhibited obvious differences. The color change of WO 3 nanowires and H–D exchange experiments suggest that when H 2 was introduced into the reaction system, hydrogen spillover can occur and the strength of hydrogen spillover decreases with increasing distance, which is in good accordance with the TPR result. Moreover, isotope-labeling experiments demonstrate that the active hydrogen species are not directly involved in the oxidation of organic substrates. For the catalyst with enhanced selectivity, the CoO x –Pt distance (several nanometers) is comparable to the distance of hydrogen spillover on Al 2 O 3 , implying that the controllable hydrogen spillover is responsible for the enhanced selectivity. The in situ XAFS results further confirm the explanation. It clearly reveals that the electronic structures of cobalt species during the epoxidation reaction can be successfully modulated through controlling the hydrogen spillover distance. For CoO x /50Al 2 O 3 /Pt in H 2 -TBHP condition, the cobalt species are reduced to a lower oxidation state, while for CoO x /50Al 2 O 3 in TBHP condition and CoO x /100Al 2 O 3 /Pt in H 2 -TBHP condition, the cobalt species are oxidized to a higher oxidation state. For the epoxidation reaction, one common understanding of the reaction mechanism is recognized that catalysts affect the reactions by bonding of oxygen to the metal [51] , [52] , [53] , [54] . The electronic structure of catalyst at reaction conditions affects the strength of the Co–O bond in the catalyst, which further determines the selectivity of epoxides. In addition to hydrogen spillover on the Al 2 O 3 support, other possible migration mechanisms of active hydrogen species, including carbon impurities and water-assisted H shuttling, are also considered. Carbon impurities are proposed as an alternative hydrogen migration path on nonreducible support [16] . Water-assisted H shuttling can accelerate proton transfer and is proposed to explain the enhanced performance observed in the presence of water for hydrogenation reactions [55] , [56] . However, the distance of hydrogen spillover on carbon species is far beyond the range of several nanometers [11] , [24] . Similarly, hydrogen shuttling is a remote promotional effect [57] . These mechanisms cannot fit our catalytic results well. Based on all above results, it can be concluded that the enhanced selectivity is attributed to the introduction of controllable hydrogen spillover, which is further confirmed by the H 2 pulse experiments. In the presence of controllable hydrogen spillover, cobalt species with a lower valence state are more beneficial for enhanced catalytic selectivity, as shown in Fig. 6e . Based on the successful demonstration of in-situ tailoring of Co valence by hydrogen spillover, we can expect that the selectivity can also be changed over a CoO x Pt/50Al 2 O 3 catalyst with the closely contacted Pt and CoO x (Supplementary Fig. 21 ) due to the effect of hydrogen spillover. As expected, the SO selectivity of CoO x Pt/50Al 2 O 3 in the H 2 -TBHP condition is also increased compared to that in the TBHP condition (Supplementary Table 9 ). This further confirms that the introduction of controllable hydrogen spillover is responsible for the enhanced selectivity. The strategy by introducing controllable hydrogen spillover into reaction was also successfully applied to the epoxidation of a variety of styrene derivatives (Table 3 ). In all cases, CoO x /50Al 2 O 3 /Pt exhibits greatly enhanced selectivities (up to over 90%) via the introduction of controllable hydrogen spillover. Further, the Pt/50Al 2 O 3 /CoO x (Supplementary Fig. 22 ), which was produced by exchanging the deposition sequences of Pt and CoO x nanoparticles, also exhibits enhanced SO selectivity through the introduction of controllable hydrogen spillover (Supplementary Table 10 ). In addition to cobalt catalysts, iron catalysts were also applied for styrene epoxidation. The SO selectivity of FeO x /50Al 2 O 3 /Pt in the H 2 -TBHP condition is higher than that of FeO x /50Al 2 O 3 in the TBHP condition (Supplementary Fig. 23 ). These results demonstrate that the introduction of controllable hydrogen spillover for enhanced selectivity is a general method. Table 3 Catalytic epoxidation of styrene derivatives in different conditions a . Full size table In summary, we have demonstrated a strategy, involving the introduction of controllable hydrogen spillover to the styrene epoxidation reaction to in situ tune the electronic structure of cobalt species for enhanced SO selectivity. The strength of hydrogen spillover from Pt nanoparticles to CoO x was tuned by altering the thickness (ALD cycles) of the separating Al 2 O 3 layer. When the thickness of the Al 2 O 3 layer was 7 nm, the catalyst (CoO x /50Al 2 O 3 /Pt) in the H 2 -TBHP condition exhibited significantly enhanced SO selectivity (over 20%) compared with the CoO x /50Al 2 O 3 catalyst in the TBHP condition. Our method of in situ electronic structure regulation, achieved through controllable hydrogen spillover, can be used for other catalytic reactions. Synthesis of 50Al 2 O 3 /Pt catalysts The synthesis of CNCs and the ALD process can be found in the Supplementary Methods. CNCs were firstly deposited with Pt nanoparticles (20 cycles) and then coated with an Al 2 O 3 layer (50 cycles) by ALD, producing 50Al 2 O 3 /Pt/CNCs. The 50Al 2 O 3 /Pt/CNCs were calcinated at 500 °C for 1 h in air to remove the CNC templates, obtaining 50Al 2 O 3 /Pt catalysts. Synthesis of CoO x /50Al 2 O 3 catalysts CNCs were firstly coated with an Al 2 O 3 layer (50 cycles) by ALD producing Al 2 O 3 /CNCs, which were calcinated at 500 °C for 1 h in air. Then the obtained hollow Al 2 O 3 nanotubes were deposited with CoO x nanoparticles (35 cycles) by ALD, obtaining CoO x /50Al 2 O 3 catalysts. Synthesis of CoO x / y Al 2 O 3 /Pt catalysts CNCs were firstly deposited with Pt nanoparticles and then coated with an Al 2 O 3 layer ( y = 35, 50, 65, 80, 100, 300) by ALD. After Al 2 O 3 deposition, CNCs were completely enclosed by compact ALD Al 2 O 3 . The obtained samples were calcinated at 500 °C for 1 h in air and subsequently coated with CoO x nanoparticles (35 cycles) by ALD, obtaining CoO x / y Al 2 O 3 /Pt. Synthesis of CoO x Pt/50Al 2 O 3 catalysts The hollow Al 2 O 3 nanotubes prepared by the above method were deposited with Pt (20 cycles) and CoO x nanoparticles (35 cycles) by ALD, obtaining CoO x Pt/50Al 2 O 3 catalysts. Synthesis of Pt/50Al 2 O 3 /CoO x catalysts CNCs were firstly deposited with CoO x nanoparticles (35 cycles) and then coated with an Al 2 O 3 layer (50 cycles) by ALD. The obtained samples were calcinated at 500 °C for 1 h in air and subsequently coated with Pt nanoparticles (20 cycles) by ALD, obtaining Pt/50Al 2 O 3 /CoO x . Synthesis of FeO x /50Al 2 O 3 and FeO x /50Al 2 O 3 /Pt catalysts The hollow Al 2 O 3 nanotubes and the 50Al 2 O 3 /Pt catalysts prepared by the above method were deposited with FeO x nanoparticles (70 cycles) by ALD, obtaining FeO x /50Al 2 O 3 and FeO x /50Al 2 O 3 /Pt catalysts, respectively. Catalyst characterizations FIB based on high-brightness Ga liquid-metal ion sources was recorded in FIB-SEM instrument (LYRA3 XMH, TESCAN). Typically, CNCs were first dispersed on a Si substrate and then were deposited by Pt and Al 2 O 3 ALD. After calcination, the CoO x was deposited. Then the Si substrate with the CoO x /50Al 2 O 3 /Pt sample was transferred into the FIB-SEM system. The sample was first protected by a carbon layer. After that, a selected part of the protected CoO x /50Al 2 O 3 /Pt was lifted out of the Si substrate by FIB milling using Ga ion beam and then mounted on a TEM grid. Finally, the sample was sliced down to ~100 nm along the vertical direction of the Al 2 O 3 nanotubes by the Ga ion beam for TEM analysis. The EPR spectrums of the reaction solutions were recorded on a Bruker EMX spectrometer (EMXplus-10/12) using the following settings: frequency 9.862 GHz, sweep width 3460.0 G, time constant 60 ms, modulation frequency 100 kHz, modulation width 0.5 G, microwave power 5 mW. The spin trap N-tert-butyl-α-phenylnitrone (PBN) was added into the reaction solutions to form radical adducts (1:1 molar ratio between the spin trap and TBHP). The solutions were filtered and the spectra were obtained at room temperature (298 K), using capillary tubes with the same dimensions as those used for the recording of the spectra of the catalysts. H–D exchange was characterized by in-situ infrared (IR) spectroscopy. IR spectra were recorded with a Bruker IFS 66v/S spectrometer with a resolution of 2 cm −1 , and each spectrum is an average of 64 scans. The sample for IR spectroscopy was loaded into a diffuse reflectance infrared Fourier transform spectroscopy (DRIFTS) cell (Harrick Scientific Products, Praying MantisTM). The cell was connected to a flow system that allows recording of spectra while gases pass through and around the sample. The samples in IR cell were pretreated at 473 K for 1 h and then cooled down to 353 K in flowing He (30 mL min −1 ). After the treatment, the samples were exposed to flowing gas (H 2 at 30 mL min −1 ) at 353 K for 1 h, and then switched to flowing gas mixtures (H 2 at 15 mL min −1 , D 2 at 15 mL min −1 ) at 353 K. The spectra of H–D exchange were recorded. The ex situ and in situ XAFS were obtained on the 1W1B beamline of the Beijing Synchrotron Radiation Facility (BSRF), Institute of High Energy Physics, Chinese Academy of Sciences, and the BL14W1 beamline of the Shanghai Synchrotron Radiation Facility (SSRF), Shanghai Institute of Applied Physics, Chinese Academy of Sciences. A Si (111) double-crystal monochromator was used to reduce the harmonic component of the monochrome beam. Co foil, CoO, and Co 3 O 4 were used as reference samples and measured in transmission mode. IFEFFIT software was used to calibrate the energy scale, to correct the background signal and to normalize the intensity. The theoretical paths for Co–O and Co–Co species used for fitting three coordination shells of the experimental data were generated using the FEFF7 program. The coordination number, bond distance, Debye–Waller factor, and inner potential correction were used as variable parameters for the fitting procedures. The in-situ XANES spectrum was simulated by a linear combination of the ex-situ spectrum of the as-prepared catalyst and the spectra of reference samples (Co 3 O 4 and CoO). The following formula was used: (in situ XANES) = f 1 ·(ex situ XANES) + f 2 ·(XANES of Co 3 O 4 ) + f 3 ·(XANES of CoO), where f 1 , f 2 , and f 3 are the fractions of the as-prepared catalyst, Co 3 O 4 and CoO, respectively. The other characterizations are provided in the Supplementary Methods. Catalytic activity measurements Styrene epoxidation reactions over the catalysts were carried out in a 50 ml three-necked round bottom flask equipped with a magnetic stirrer in an oil bath. A mixture of catalysts with the same CoO x content, 20 ml acetonitrile, 3.5 mmol styrene, and 7 mmol TBHP (70% TBHP in water) was introduced into the reaction vessel. Then, the reaction mixture was magnetically stirred and heated to 80 °C at atmospheric pressure. When H 2 was introduced into the reaction, the vessel was purged with purified hydrogen to remove the air at atmospheric pressure, and then was completely sealed with rubber plugs. Heating the reaction system to 80 °C, styrene was injected through needle tube. After reaction for 8 h, the reaction mixture was separated and the liquid products collected were analyzed by gas chromatography–mass spectrometry (GC–MS, Agilent Technologies 7890A-5795C) with a capillary column (HP-5, 30 m × 25 mm × 0.25 μm). Free radical capture experiments were carried out by adding 2 mmol quenchers (BHT) into the reaction system after 1 h reaction. H 2 pulse experiments were carried out in a 50 ml three-necked round bottom flask with alternating pulse of H 2 and air. When the reaction atmosphere was displaced, the heating was stopped and each displaced process was maintained for 10 min with the gas flow rate of 30 sccm. Note that before each pulse, air or H 2 was purged by inert gas nitrogen to ensure the safety. After displacement, the vessel was completely sealed and continued to be heated. The samples were collected every hour, and the reaction atmosphere was displaced every 2 h. Mixing hydrogen with an oxidant, in principle, may be not safe. In this paper, the risks are very minor considering mild reaction condition (low reaction temperature, atmospheric pressure, a small amount of H 2 (30  ml), and a round bottom flask sealed with rubber plugs). If readers attempt to repeat it, please refer to the detailed experiment process in the section of “Catalytic activity measurements”.